Ultrafast X-ray Auger probing of photoexcited molecular dynamics Molecules can efficiently and selectively convert light energy into other degrees of freedom. Disentangling the underlying ultrafast motion of electrons and nuclei of the photoexcited molecule presents a challenge to current spectroscopic approaches. Here we explore the photoexcited dynamics of molecules by an interaction with an ultrafast X-ray pulse creating a highly localized core hole that decays via Auger emission. We discover that the Auger spectrum as a function of photoexcitation—X-ray-probe delay contains valuable information about the nuclear and electronic degrees of freedom from an element-specific point of view. For the nucleobase thymine, the oxygen Auger spectrum shifts towards high kinetic energies, resulting from a particular C–O bond stretch in the ππ* photoexcited state. A subsequent shift of the Auger spectrum towards lower kinetic energies displays the electronic relaxation of the initial photoexcited state within 200 fs. Ab-initio simulations reinforce our interpretation and indicate an electronic decay to the nπ* state. Some molecules have the ability to selectively and efficiently convert light into other forms of energy such as heat and charge separation, or store it in altered chemical bonds. These processes often require transitions between the multiple electronic states of the molecule, proceeding through violations of the Born–Oppenheimer approximation (BOA) [1] . The BOA allows the separation of electronic and nuclear degrees of freedom and is an important tool for the prediction of molecular properties. Non-BOA transitions between different electronic states pose challenges to theory and experiment; they are difficult to model, they proceed on an ultrafast timescale and prominently occur at so-called conical intersections (CIs) of electronic potential energy surfaces [2] , [3] , [4] (see Fig. 1a ). The theory of non-BOA dynamics has advanced significantly over the last two decades, but challenges in the simulation of photoexcited electronic structure and non-BOA dynamics persist, even for the high-level methods employed in isolated molecules [4] , [5] , [6] . Experiments on non-BOA dynamics in isolated molecules typically use ultrafast optical pulses for probing molecular dynamics, utilizing transitions between mostly delocalized electrons [7] , [8] , [9] . 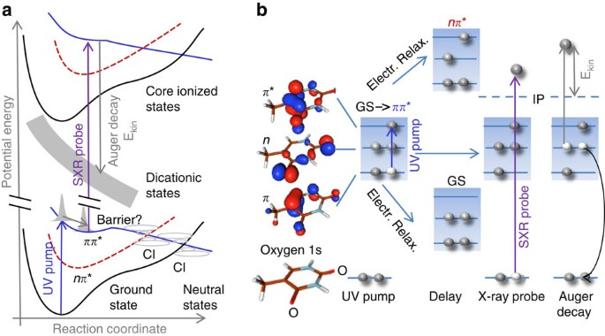Figure 1: Potential energy surfaces and ultrafast Auger probe scheme. (a) Sketch illustrating general features of photoexcited molecular states. After a light-induced electronic transition, a nuclear wavepacket is driven by gradients in the potential energy surface (blue) towards regions containing conical intersections (CIs), allowing for ultrafast electronic transitions to lower electronic states (red and black) under violation of the Born–Oppenheimer approximation. The electronic relaxation of the photoexcited population can be intercepted by reaction barriers between the initial photoexcited reaction coordinate and CI region. For the particular case of thymine, the UV excitation (pump) pulse excites a wavepacket on theππ* state and CIs connect tonπ* and ground state (GS). The topology of theππ* state controls the speed of electronic relaxation and the height of the sketched barrier is currently a matter of debate. The soft X-ray probing is shown by a transition to core-ionized molecular potential energy surfaces, from which the Auger decay proceeds to a manifold of dicationic states. The potential energy difference between core ionized and dicationic state determines the kinetic energy of the Auger electron. (b) Ultrafast Auger probing applied to thymine photoprotection. The images on the left side show theπ, nandπ* molecular valence orbitals. The oxygen 1s orbitals, in which the core hole can be created, are highly localized at one of the marked two oxygen sites. Theπandnorbitals are both doubly occupied in the ground state configuration. The UV pump pulse promotes an electron from aπorbital to aπ* orbital, giving rise to the chemically reactiveππ* state. We probe the electronic valence state by a delayed soft X-ray (SXR) probe pulse creating a core hole and inducing Auger decay. The emitted Auger electrons carry information about the valence electronic state at the core-hole position (oxygen in our case). Figure 1: Potential energy surfaces and ultrafast Auger probe scheme. ( a ) Sketch illustrating general features of photoexcited molecular states. After a light-induced electronic transition, a nuclear wavepacket is driven by gradients in the potential energy surface (blue) towards regions containing conical intersections (CIs), allowing for ultrafast electronic transitions to lower electronic states (red and black) under violation of the Born–Oppenheimer approximation. The electronic relaxation of the photoexcited population can be intercepted by reaction barriers between the initial photoexcited reaction coordinate and CI region. For the particular case of thymine, the UV excitation (pump) pulse excites a wavepacket on the ππ * state and CIs connect to n π * and ground state (GS). The topology of the ππ * state controls the speed of electronic relaxation and the height of the sketched barrier is currently a matter of debate. The soft X-ray probing is shown by a transition to core-ionized molecular potential energy surfaces, from which the Auger decay proceeds to a manifold of dicationic states. The potential energy difference between core ionized and dicationic state determines the kinetic energy of the Auger electron. ( b ) Ultrafast Auger probing applied to thymine photoprotection. The images on the left side show the π , n and π * molecular valence orbitals. The oxygen 1s orbitals, in which the core hole can be created, are highly localized at one of the marked two oxygen sites. The π and n orbitals are both doubly occupied in the ground state configuration. The UV pump pulse promotes an electron from a π orbital to a π * orbital, giving rise to the chemically reactive ππ * state. We probe the electronic valence state by a delayed soft X-ray (SXR) probe pulse creating a core hole and inducing Auger decay. The emitted Auger electrons carry information about the valence electronic state at the core-hole position (oxygen in our case). Full size image In this work, we show that element and site-specific probing by soft X-ray (SXR) pulses in combination with Auger electron detection can resolve non-BOA processes in isolated molecules, even for cases that are not easily detected by traditional ultrafast experiments. We perform ultrafast Auger probing of photoinduced non-BOA dynamics in thymine at the LINAC coherent light source (LCLS). We selectively probe the initial elongation of a C–O bond after molecular photoexcitation, which is displayed by a shift of the Auger spectrum to higher kinetic energies. From a subsequent shift to lower kinetic energies we deduce an initial photoexcited state lifetime of 200 fs. Our results demonstrate that ultrafast Auger probing is able to distinguish between nuclear relaxation and non-BOA electronic transitions. Using the Auger spectrum to probe photoexcited dynamics is applicable to very dilute targets and therefore complements the method of ultrafast SXR absorption spectroscopy, which is ideally suited for condensed phase high-density targets [10] , [11] . Strategy for the ultrafast X-ray probe In our experiment, performed at the LCLS, the SXR probe pulse ionizes a highly localized oxygen 1s electron after the molecule has been excited by an ultrashort ultraviolet pulse, which has changed the valence electronic occupation (see Fig. 1b ). The core-ionized state promptly decays to a dicationic state by filling the core hole with a valence electron and emitting an Auger electron (see Fig. 1 ). The Auger electron kinetic energy is analysed using a spectrometer as a function of pump-probe delay (see Methods). Ultrafast Auger probing has several compelling advantages for elucidating non-BOA dynamics: first, SXRs with energies of several eV above the absorption edge are capable of core-ionizing the molecule at any nuclear geometry. Thus the signal strength does not decrease due to reduced Franck–Condon overlap upon vibrational relaxation. The latter can be problematic in other ultrafast pump-probe spectroscopies using optical pulses. Second, the core electron-binding energies as well as the Auger kinetic energies differ vastly for different elements and sites within a molecule. This allows us to observe the nuclear as well as the electronic dynamics of the molecule from a highly local point of view. Similar to infrared spectroscopy we can monitor the motion of certain bonds within the molecule, but in addition we obtain information on the molecular electronic state. Third, as we will show here, the nuclear and electronic relaxation cause distinct transient shifts in the Auger spectra, aiding the interpretation. Importantly, Auger spectra are insensitive to the strong spectral fluctuations that are typical in self-amplified spontaneous emission X-ray free-electron laser sources, which are currently the most common ultrashort SXR laser sources [12] . The difficulties of resolving excited state molecular dynamics through pump-probe experiments are illustrated using a sketch of potential energy surfaces along a one-dimensional reaction coordinate in Fig. 1a . A wavepacket, which is launched in the Franck–Condon region of a neutral photoexcited state (blue), follows potential gradients and immediately starts to relax along a nuclear coordinate. It reaches regions with CIs that connect to other electronic states (red and black), offering an ultrafast electronic relaxation route. Along the path from the Franck–Condon to the CI region other features, such as reaction barriers, may be encountered. Distinguishing the ultrafast nuclear relaxation on the initially photoexcited state from electronic relaxation presents a challenge to the interpretation of ultrafast measurements with optical pulses, because both can lead to a transient signal decay. Application for thymine This prototypical difficulty is exemplified with the case of the nucleobase thymine. Thymine shows an electronic relaxation process out of the photoexcited π π * state (blue). This relaxation contributes to the protection of DNA from damaging ultraviolet-induced dimerization [13] , [14] . Previous time-resolved ion [15] , [16] , [17] and photoelectron measurements [18] in isolated molecules aimed at attributing a time constant to the electronic relaxation. They all showed a very short, ~\n100 fs, decay constant followed by additional 5–7 ps decay [15] , [16] , [17] , [18] . The time constants are generally consistent with calculations of the potential energy surface [19] , [20] , [21] , [22] , [23] . However, the assignment of the transients to electronic or nuclear relaxation varies among theoretical approaches, as it depends strongly on the reaction path and reaction barrier in the π π * state, which is particularly sensitive to the chosen quantum chemical methodology. Approaches based on linear interpolation [21] or minimal energy paths [22] predict a barrierless and thus very fast decay to the electronic ground state not involving any C–O bond stretch. This suggests an interpretation of the fastest time constant as electronic relaxation. A second, so-called indirect path [23] was suggested to compete with the direct ultrafast electronic relaxation to the ground state. The full dynamics simulation [19] predicts an initial ultrafast nuclear relaxation into the π π * state minimum involving the C(4)–O(8) stretch. The population is then trapped for picoseconds behind a reaction barrier. These results have been extended to much longer timescales stating that molecular population transfers into the n π * state with a picoseconds time constant [20] . This suggests an interpretation of the 100 fs constant as a nuclear relaxation. The thymine photochemistry clearly represents a difficult case for theory and experiment, motivating further ultrafast experimental studies. The SXR pulses used in our investigation are capable of core-ionizing the molecule in any nuclear geometry and thus the integrated Auger signal persists upon nuclear relaxation on the π π * state. Moreover, we will show that Auger spectroscopy allows for experimental separation of electronic and nuclear relaxation. Nuclear relaxation on π π * includes an elongation of the C(4)–O(8) bond close to the methyl group (see Fig. 2 ), which is intuitively clear from the π * orbital shape having a node on this C–O bond (see Fig. 1b orbital scheme). We will show that this elongation results in a blueshift of X-ray-induced Auger spectra. In contrast, electronic relaxation from the π π * state to the n π * or the ground state manifests itself as a shift towards lower kinetic energies (see below). 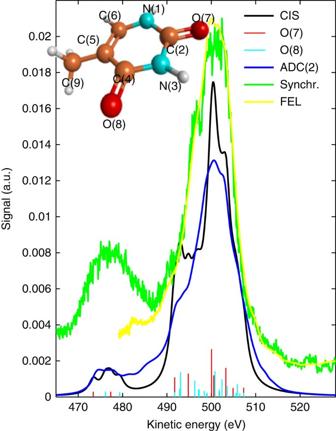Figure 2: Ground state Auger spectrum. Comparison of experimental and theoretical ground-state Auger spectra for thymine. The green and yellow curves are data taken at the Advanced Light Source (ALS) synchrotron and the LCLS free-electron laser, respectively, and are offset in intensity from the theory. The magnetic bottle spectrometer employed for the FEL measurements used a retardation voltage of 470 eV leading to a reduction in transmission for the lower kinetic energy range until about 487 eV. The ADC(2) calculations (blue) as well as the CK-CIS simulations (black) are explained in theSupplementary Information, they reproduce the essential features of the experiment and are in general agreement. The lines from the CK-CIS calculations are shown by sticks reflecting the Auger rate from distinct valence orbitals that have a large spatial overlap with the oxygen 1s core orbitals. The sticks for the O(7) atom (red) and the O(8) atom (blue) produce similar Auger spectra (see alsoSupplementary Tables 1 and 2). The inset shows the molecular geometry with the number convention used for its atoms. Figure 2: Ground state Auger spectrum. Comparison of experimental and theoretical ground-state Auger spectra for thymine. The green and yellow curves are data taken at the Advanced Light Source (ALS) synchrotron and the LCLS free-electron laser, respectively, and are offset in intensity from the theory. The magnetic bottle spectrometer employed for the FEL measurements used a retardation voltage of 470 eV leading to a reduction in transmission for the lower kinetic energy range until about 487 eV. The ADC(2) calculations (blue) as well as the CK-CIS simulations (black) are explained in the Supplementary Information , they reproduce the essential features of the experiment and are in general agreement. The lines from the CK-CIS calculations are shown by sticks reflecting the Auger rate from distinct valence orbitals that have a large spatial overlap with the oxygen 1s core orbitals. The sticks for the O(7) atom (red) and the O(8) atom (blue) produce similar Auger spectra (see also Supplementary Tables 1 and 2 ). The inset shows the molecular geometry with the number convention used for its atoms. Full size image Ground state Auger spectra Figure 2 shows a comparison of experimental (free-electron laser with synchrotron data) and simulated oxygen Auger 1s electron spectra for thymine in the electronic ground state. The theoretical analysis is described in Supplementary Note 1 . The high-level algebraic diagrammatic construction (ADC(2)) [24] , [25] method simulates the observed features well. For excited states, the ADC(2) method is unfeasible, and we developed a lower-level approach based on the complex Kohn [26] and configuration interaction singles (CK-CIS) method [27] . To further simplify our approach, we concentrate only on the strongest Auger transitions (shown as lines), which are broadened by spectrometer and lifetime limitations. Although the CK-CIS method is expected to be less accurate than ADC(2), it has the advantage of providing access to features of the photoexcited-state Auger decay. The molecular valence orbitals that are strongly localized at the core-ionized oxygen site dominate the Auger decay features calculated with the ADC(2) and CK-CIS methods ( Supplementary Tables 1 and 2 ). This is the underlying basis of Auger decay element sensitivity. Transient Auger spectra The change of the Auger spectrum following ultraviolet excitation is shown as difference spectra in Fig. 3a as a function of pump-probe delay. The subtraction of unexcited spectra from ultraviolet-excited spectra reveals the change between the unexcited and excited molecule (see the Methods section). 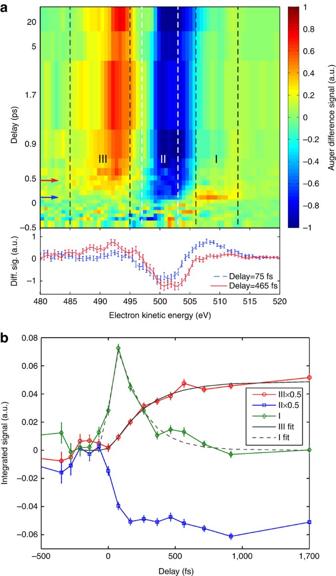Figure 3: Ultrafast Auger probe data. (a) Difference Auger spectra with and without UV excitation as function of Auger electron kinetic energy and time delay between UV pump and soft X-ray probe pulse. The colour encodes the difference in Auger yield: blue: UV induces less Auger decay, red: UV induces more Auger decay. The kinetic energy axis is divided in three ranges I (506–513 eV), II (497–503 eV) and III (485–495 eV). A time resolution around 70 fs has been achieved by single shot delay measurements34and subsequent resorting of our data. Note the non-equidistant time intervals. The bottom part shows difference spectra at two different delays marked by the arrows (75 fs dashed blue and 465 fs solid red). (b) Integrations over kinetic energy range in (a) scaled by a factor as given in the legend. The grey lines show the fit described inSupplementary Note 2. Figure 3b shows the integrated signal in the kinetic energy intervals (I, II and III) for different delays. The fastest features are a decrease in region II accompanied by a rise in region I. This reflects a shift of the whole Auger band towards higher Auger kinetic energies due to ultraviolet excitation. The immediate appearance of this modulation in regions I and II reflect the creation of a wavepacket in the π π * excited state by the ultraviolet pulse. Figure 3: Ultrafast Auger probe data. ( a ) Difference Auger spectra with and without UV excitation as function of Auger electron kinetic energy and time delay between UV pump and soft X-ray probe pulse. The colour encodes the difference in Auger yield: blue: UV induces less Auger decay, red: UV induces more Auger decay. The kinetic energy axis is divided in three ranges I (506–513 eV), II (497–503 eV) and III (485–495 eV). A time resolution around 70 fs has been achieved by single shot delay measurements [34] and subsequent resorting of our data. Note the non-equidistant time intervals. The bottom part shows difference spectra at two different delays marked by the arrows (75 fs dashed blue and 465 fs solid red). ( b ) Integrations over kinetic energy range in ( a ) scaled by a factor as given in the legend. The grey lines show the fit described in Supplementary Note 2 . Full size image The immediate blueshift of the Auger spectrum after photoexcitation is connected to nuclear relaxation dynamics. As pointed out above, probing the oxygen Auger decay gives us the advantage of monitoring nuclear and electronic dynamics of bonds in the vicinity of oxygen atoms, which are two C–O bonds for thymine. A stretch in these bonds leads to a blueshift in the Auger spectrum. This can be understood from electrostatic considerations with the help of Fig. 1a . The final states in the Auger decay with two valence holes (dicationic states given in grey) are strongly repulsive owing to some unscreened nuclear repulsion. They have lower bond strength and therefore a lowered electronic energy for increasing C–O bond lengths (see Fig. 1a ). Thus the energy difference between the core-ionized state and the very repulsive dicationic final state increases along the C–O stretch, which increases with the reaction coordinate. This effect leads to a blueshifted Auger spectrum. Resolving the C–O bond motion in time as a continuous energy shift would require better time resolution for our signal-to-noise levels. This argument is supported by CK-CIS simulations, as shown in Fig. 4a,b depicting Auger spectra for the ground state, the π π * state at the Franck–Condon and π π * minimum geometries. The π π * state at the Franck–Condon geometry is slightly shifted blue with respect to the ground state and an even larger shift occurs at the π π * minimum. The CK-CIS Auger spectrum can be separated according to which of the oxygen atoms was core-excited. Remarkably, only the spectrum arising from O(8) (thin solid blue) shows major changes upon excited state relaxation. The O(7) (dashed blue line) spectrum is rather static since the C(2)–O(7) bond does not change as a consequence of photoexcitation. The C(4)–O(8) bond elongates by 15% as the molecule changes from the Franck–Condon nuclear geometry to the π π * state minimum [19] , [20] . This fast nuclear relaxation results in a large Auger blueshift comparable to the shift observed in the experimental difference spectrum measured for 75 fs delay ( Fig. 4e ). This confirms that nuclear relaxation including the C(4)–O(8) elongation out of the Frank–Condon region leads to a consistent shift towards higher kinetic energies, just as qualitatively expected from experimental considerations. 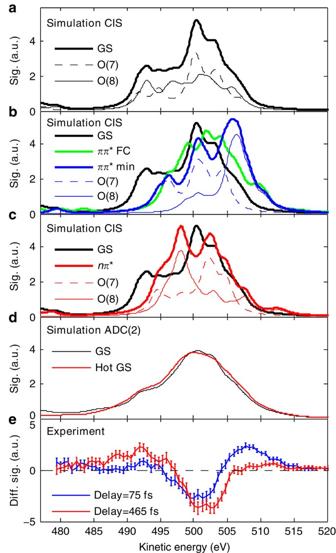Figure 4: Ultrafast Auger probe simulations. Calculated Auger decay spectra using the CK-CIS method (seeSupplementary Note 1) for the ground-state GS, thenπ* andππ* (a–c), states (seeSupplementary Tables 1–6for more information on prominent Auger decay features). (a) The ground-state Auger decay is calculated at its minimum energy geometry and corresponds to the Auger decay of a non-UV excited molecule. (b) Theππ* state is evaluated at the Frank–Condon geometry and theππ* minimum geometry according to ref.19. While the spectrum of O(7) does not shift with respect to the ground state, the O(8) spectrum shifts blue in theππ* minimum because of the C(4)-O(8) stretch. (c) The simulation predicts a redshift fornπ* states, which once more is only due to the O(8) spectrum. Other geometries on the respective state confirm the trend (seeSupplementary Fig. 1). The vibrationally hot electronic ground state in (d) calculated by the ADC(2) method via averaging different nuclear geometries (seeSupplementary Fig. 2) broadens the Auger spectrum with respect to the the ADC(2) simulation of the ‘cold’ ground state for reference. (e) Experimental difference spectra cut at two different times fromFig. 2a(lower part) indicating a shift towards higher kinetic energy at early times and lower kinetic energies later. Figure 4: Ultrafast Auger probe simulations. Calculated Auger decay spectra using the CK-CIS method (see Supplementary Note 1 ) for the ground-state GS, the n π * and π π * ( a – c ), states (see Supplementary Tables 1–6 for more information on prominent Auger decay features). ( a ) The ground-state Auger decay is calculated at its minimum energy geometry and corresponds to the Auger decay of a non-UV excited molecule. ( b ) The π π * state is evaluated at the Frank–Condon geometry and the π π * minimum geometry according to ref. 19 . While the spectrum of O(7) does not shift with respect to the ground state, the O(8) spectrum shifts blue in the π π * minimum because of the C(4)-O(8) stretch. ( c ) The simulation predicts a redshift for n π * states, which once more is only due to the O(8) spectrum. Other geometries on the respective state confirm the trend (see Supplementary Fig. 1 ). The vibrationally hot electronic ground state in ( d ) calculated by the ADC(2) method via averaging different nuclear geometries (see Supplementary Fig. 2 ) broadens the Auger spectrum with respect to the the ADC(2) simulation of the ‘cold’ ground state for reference. ( e ) Experimental difference spectra cut at two different times from Fig. 2a (lower part) indicating a shift towards higher kinetic energy at early times and lower kinetic energies later. Full size image We observe a decrease in region I with a 200-fs time constant together with a rise in region III, indicating a population transfer to an excited state with lower Auger kinetic energies. This is contrary to the nuclear relaxation trend described above. The observed experimental shift therefore disagrees with further nuclear relaxation and indicates an electronic relaxation. This fast electronic decay of the π π * state must occur unimpeded by any significant reaction barrier within the relaxation path. We cannot exclude that potential maxima exist on the side of the path and are circumvented by the molecular wavepacket. These barriers, however, cannot be directly measured via population trapping. We now concentrate on the interpretation of the signal in region III in terms of product states. A return of photoexcited population to the vibrationally hot ground state as well as population of the dark n π * state is possible and was controversially discussed in the theoretical literature [19] , [20] , [21] , [22] , [23] . The simulated n π * spectrum (red line, Fig. 4c ) shows a shift of its maximum into spectral region III, in agreement with our experimental observations (the shift is consistent for different nuclear geometries, see Supplementary Fig. 1 ). The simulated hot ground-state spectrum in Fig. 4d shows a rather symmetric broadening owing to the sampling over different nuclear geometries (see Supplementary Fig. 2 ). Furthermore, its modulation is shallow compared with that in the electronically excited states, indicating a low sensitivity of our experiment towards this state. We point out that the hot ground state was sampled with a reduced set of geometries owing to the computational effort associated with the chosen ADC(2) method. On the basis of the comparison of our experimental data with these preliminary theoretical results, we attribute the increase in region III to the population of the n π * state. We now compare the measured time constants and our interpretation to literature data of the thymine model system. Short decay constants on the order of 100 fs have been documented in the optical pump-probe literature [15] , [16] , [17] , [18] and were interpreted either as nuclear relaxation on the π π * state or electronic relaxation out of this state. The SXR experiments described here distinguish between nuclear and electronic relaxation and we can interpret the 200-fs decrease in region I as an electronic reduction of the π π * population. The fast decay of a majority of the π π * state population is in agreement with some previous theoretical calculations of the π π * potential energy surface [21] , [22] , [23] . We are not able to resolve the 100-fs process observed in optical experiments, but it is most likely hidden in the blueshift due to nuclear relaxation out of the π π * Franck–Condon window. Several simulations point towards relaxation to a hot ground state within a few 100 fs [21] , [22] , [23] , which was confirmed in liquid phase [28] . Owing to reduced Auger sensitivity to this state, we cannot discern the importance of this relaxation channel from our measurement. Our experimental transients together with Auger simulations of the n π * state, however, point towards a 200–300-fs filling of the n π * state. Dynamical simulations predict a several ps timescale [19] , [20] for this process and the discrepancy might originate from an overestimated reaction barrier [21] , [23] . In order to show excited state fluorescence as measured in liquid phase according to ref. 29 , some molecular population must be trapped behind a reaction barrier, but we assume that our experimental signal-to-noise ratio is not good enough to deduce such detailed information. In summary, we have demonstrated a new method for accessing the photoinduced dynamics on excited states of isolated molecules. The ultrafast Auger probe technique is particularly well suited to distinguish ultrafast nuclear and electronic relaxation with high local sensitivity. A particular advantage of the ultrafast Auger probe method lies in different spectral features for nuclear and electronic relaxation, which allows a new perspective on dynamics. We have found a 200-fs electronic relaxation of a majority of the photoexcited π π * state in thymine, and thus conclude that under the conditions in this experiment the majority of the excited-state population is not efficiently trapped by an excited-state reaction barrier as previously suggested. Tuning the X-ray wavelength into the resonance region could result in site-specific resolution of molecular dynamics in the future. The ultrafast Auger probe method is ideal for dilute quantum systems, and complements the now established method of ultrafast SXR absorption spectroscopy applicable to high-density targets [10] , [11] . The method makes optimal use of X-rays sources with short pulse duration and high fluence. Such sources are now available owing to the development of free-electron lasers such as LCLS [30] , FLASH [31] and SACLA [32] . Setups Our experiments are performed at the LCLS at SLAC National Accelerator Laboratory and at the Advanced Light Source at Lawrence Berkeley National Laboratory. At LCLS, our experiment took place in the high field physics chamber of the atomic, molecular and optical science instrument [33] . Molecules evaporated by a 140-°C hot oven were guided to the photon interaction region through a 900-micron diameter, 40-mm-long capillary. Measurements on the beam ex situ gave an estimated sample density of 10 11 molecules cm −3 at the exit of the capillary and a molecular beam opening angle in the range of 10°. The background pressure was in the 10 −9 mbar range, corresponding to particle densities that are 3–4 orders of magnitude below the thymine density in the interaction region. The molecules were first irradiated by a ultraviolet pulse of 266 nm wavelength having a duration of 70 fs. After a time delay in the femtosecond-to-picosecond domain, the photoexcited molecules were exposed to a SXR pulse with a photon energy of 565 eV and an estimated duration from 50 to 80 fs. The SXR pulses had a spectral jitter and bandwidth of about 0.25–0.5%. The Auger measurements were not sensitive to the spectral jitter. The relative delay between ultraviolet and SXR pulses also jittered from shot to shot, giving at best a temporal resolution near 250 fs. We markedly increase our temporal resolution to 70 fs by characterizing the jitter with a single shot, X-ray optical cross-correlator that measures and re-sorts the shots according to delay [34] . The ultraviolet pump pulse was focused to a ~\n70-micron spot, estimated from a microscope image of a yttrium aluminium garnet screen in the interaction region. The X-rays were focused more tightly than the ultraviolet. The energy of the ultraviolet pulses and the X-ray pulses were chosen to avoid nonlinear effects that can result in the production of double core holes [35] , [36] , [37] , [38] or two-photon ionization [39] , thereby changing the spectrum. This was checked by observing the spectra during a systematic scan of both pulse energies independently. Since the multiphoton ultraviolet excitation lead to molecular fragmentation, it was easy to confirm the low excitation limit. The SXR pulse creates 1s core holes in carbon, nitrogen and oxygen inside the molecule according to their relative absorption cross-sections. The photoelectrons were discarded, since their energy fluctuated strongly with the LCLS spectral jitter. Instead we analysed the Auger electrons around 500 eV kinetic energy, which are exclusively ejected by an O 1s core hole decay. The electrons were funneled towards a 2-m-long flight tube by a strong permanent magnet. They encounter a retardation of 470 V and hit an microchannel plate detector to measure their time of flight, which is then converted to kinetic energy. The spectrometer was designed as a magnetic bottle [40] ; however, we turned the solenoid in the flight tube off to increase the spectral resolution. The presence of the permanent magnet provided a high spatial sensitivity on the intersection region between the pump and probe pulse. With this setup, we were able to distinguish lines spaced by 2 eV in the Xe-MNN-Auger spectrum [41] , which also served as our calibration standard. The polarizations of the ultraviolet and SXR pulses were aligned with the flight tube symmetry axis. At the Advanced Light Source, we used beamline 8 to record Auger spectra of unexcited molecules at variable photon energies for N, C and O core hole decay. The kinetic energy of the Auger spectra was measured with a hemispherical analyzer whose axis was aligned to 56° with respect to the SXR polarization. The molecules were evaporated at similar temperatures to the LCLS experiments into a gas cell flanged onto the analyzer. Difference signal interpretation Assuming a fraction f of the molecules were excited by the ultraviolet pulse, the difference signal is given as Signal(UV on )−Signal(UV off )=Signal GS (1− f )+Signal ES f −Signal GS = f (Signal ES −Signal GS ), where the subscripts GS and ES refer to the ground and photoexcited molecular states, respectively. The Signal(UV on ) and Signal(UV off ) spectra are the mean of the single shot spectra that fall into a selected delay interval; the error is the s.e. of this mean. How to cite this article: McFarland, B. K. et al. Ultrafast X-ray Auger probing of photoexcited molecular dynamics. Nat. Commun. 5:4235 doi: 10.1038/ncomms5235 (2014).